Direct cellular delivery of human proteasomes to delay tau aggregation The 26S proteasome is the primary machinery that degrades ubiquitin (Ub)-conjugated proteins, including many proteotoxic proteins implicated in neurodegeneraton. It has been suggested that the elevation of proteasomal activity is tolerable to cells and may be beneficial to prevent the accumulation of protein aggregates. Here we show that purified proteasomes can be directly transported into cells through mesoporous silica nanoparticle-mediated endocytosis. Proteasomes that are loaded onto nanoparticles through non-covalent interactions between polyhistidine tags and nickel ions fully retain their proteolytic activity. Cells treated with exogenous proteasomes are more efficient in degrading overexpressed human tau than endogenous proteasomal substrates, resulting in decreased levels of tau aggregates. Moreover, exogenous proteasome delivery significantly promotes cell survival against proteotoxic stress caused by tau and reactive oxygen species. These data demonstrate that increasing cellular proteasome activity through the direct delivery of purified proteasomes may be an effective strategy for reducing cellular levels of proteotoxic proteins. The ubiquitin–proteasome system (UPS) is a major cellular mechanism that regulates the levels of regulatory, misfolded or damaged proteins [1] , [2] . This allows cells to maintain essential physiological functions, adapt to environmental and pathological changes and control the quality of proteins [3] , [4] , [5] . The selectivity of most Ub-mediated proteolysis is mainly controlled by specific E3 Ub ligases, which recognize temporally and spatially activated degradation signals, or degrons [6] . However, it is the 26S proteasome that irreversibly degrades target substrates within its 28-subunit core particle (CP). The CP forms a complex with a 19-subunit regulatory particle (RP), which interacts with substrates' polyubiquitin chains, translocates the substrates into the CP, and deubiquitinates the polyubiquitin chains before degradation commences [7] . Due to methodological limitations and the exceptional complexity of the system, regulatory mechanisms of proteasome activity and homeostasis remain poorly understood. Overall UPS output is reportedly decreased in various neurodegenerative disorders including Alzheimer’s disease (AD). This may be linked to the age-dependent decline in proteasome activity and the accumulation of tau aggregates that reciprocally clog the proteasome’s entry pore [8] , [9] . If so, then artificially enhanced cytoplasmic proteasome activity may depress lesion formation in disease [10] , [11] . However, the contribution of proteasome-mediated clearance to tau metabolism has been contentious [8] , and so the potential of this approach has been unclear. Here we tested whether increasing proteasome activity could modulate tau metabolism by delivering purified proteasome holoenzymes directly to cells through mesoporous nanoparticles. We found that increased cellular proteasome activity stimulated tau degradation and significantly delayed tau aggregate formation in cells. These findings reveal that exogenous proteasomes may help cells cope with the proteopathic stresses implicated in various diseases. Proteasome–MSNPN complexes retain their proteolytic activities Novel mesoporous silica nanoparticles with nickel moieties (MSNPN; compound 3 in Supplementary Fig. 1 and Supplementary Note 1 ) were developed as a proteasome transporter. MSNPN were synthesized to have pore sizes between 25 and 30 nm using a pore expansion strategy [12] , [13] , which can harbour a proteasome holoenzyme molecule through non-covalent interactions with the polyhistidine (His) tag of proteasomes ( Fig. 1a ). The relatively large surface area (388 m 2 g −1 ) and pore volume (1.47 ml g −1 ) of MSNPN are also advantageous for loading and delivering proteasomes in their native conformation. Active human 26S proteasomes were effectively affinity purified from a HEK293-derived cell line stably expressing both His- and biotin-tagged β4 subunits ( Supplementary Fig. 2 ) [14] . Unlike proteasomes purified by conventional methods [10] , these proteasomes had significant amounts of USP14, a loosely associated deubiquitinating enzyme on the RP and an endogenous proteasome inhibitor [15] . 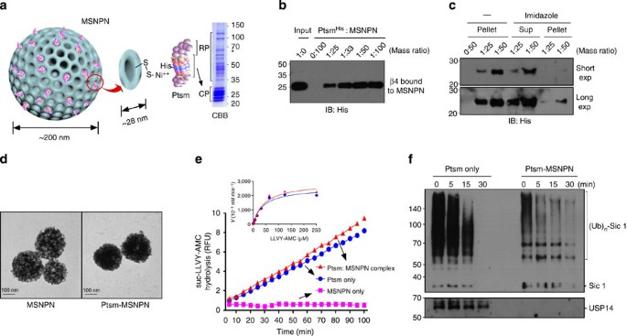Figure 1: Proteasome holoenzymes are loaded to MSNPN through non-covalent interactions and their activities are retained in the complex formation. (a) Illustration of proteasome interaction with MSNPN. Affinity-purified human proteasomes with His-tagged β4 subunits were analysed by SDS–polyacrylamide gel electrophoresis (PAGE)/Coomassie brilliant blue (CBB) staining. See alsoSupplementary Figs 2 and 3and for MSNPN and proteasome characterizations, respectively. *Proteasome-bound USP14. (b) Proteasomes were incubated with MSNPN using the indicated mass ratios. Samples were then subjected to spin-down and the pellet portions were used for SDS–PAGE and immunoblotting (IB). Input, proteasome alone with an equal amount as other proteasome–MSNPN complexes. Ptsm, 26S proteasome. (c) As inbexcept that 0.5 M imidazole was added to the reaction and the supernatant (Sup) and pellet fractions were separated for IB analysis. Short exp and long exp, short and long exposure of the blot, respectively. (d) TEM images of MSNPN and proteasome-charged MSNPN (Ptsm-MSNPN). (e) suc-LLVY-AMC hydrolysis assay using MSNPN, proteasomes, and proteasome–MSNPN complexes. The insert is the Michaelis–Menten plot of concentration-dependent suc-LLVY-AMC cleavage in the presence of proteasomes (0.4 nM) or proteasome–MSNPN complexes (1:50, 0.4 nM) for 15 min (r2>0.97). Each data point of the graphs shown represents the mean of triplicate determinations. r.f.u., relative fluorescence units. (f)In vitroproteasomal degradation assay using polyubiquitinated Sic1PY(Ub-Sic1) with T7 tags. Reactions with proteasomes or proteasome–MSNPN complexes for the indicated times were analysed by SDS–PAGE/IB using anti-T7 and anti-USP14 antibodies. Figure 1: Proteasome holoenzymes are loaded to MSNPN through non-covalent interactions and their activities are retained in the complex formation. ( a ) Illustration of proteasome interaction with MSNPN. Affinity-purified human proteasomes with His-tagged β4 subunits were analysed by SDS–polyacrylamide gel electrophoresis (PAGE)/Coomassie brilliant blue (CBB) staining. See also Supplementary Figs 2 and 3 and for MSNPN and proteasome characterizations, respectively. *Proteasome-bound USP14. ( b ) Proteasomes were incubated with MSNPN using the indicated mass ratios. Samples were then subjected to spin-down and the pellet portions were used for SDS–PAGE and immunoblotting (IB). Input, proteasome alone with an equal amount as other proteasome–MSNPN complexes. Ptsm, 26S proteasome. ( c ) As in b except that 0.5 M imidazole was added to the reaction and the supernatant (Sup) and pellet fractions were separated for IB analysis. Short exp and long exp, short and long exposure of the blot, respectively. ( d ) TEM images of MSNPN and proteasome-charged MSNPN (Ptsm-MSNPN). ( e ) suc-LLVY-AMC hydrolysis assay using MSNPN, proteasomes, and proteasome–MSNPN complexes. The insert is the Michaelis–Menten plot of concentration-dependent suc-LLVY-AMC cleavage in the presence of proteasomes (0.4 nM) or proteasome–MSNPN complexes (1:50, 0.4 nM) for 15 min ( r 2 >0.97). Each data point of the graphs shown represents the mean of triplicate determinations. r.f.u., relative fluorescence units. ( f ) In vitro proteasomal degradation assay using polyubiquitinated Sic1 PY (Ub-Sic1) with T7 tags. Reactions with proteasomes or proteasome–MSNPN complexes for the indicated times were analysed by SDS–PAGE/IB using anti-T7 and anti-USP14 antibodies. Full size image Purified proteasomes were readily loaded onto MSNPN, which appeared to be saturated at a 1:50 mass ratio (proteasome/nanoparticle), corresponding to ~37 proteasome holoenzymes charged per single nanoparticle ( Fig. 1b ). The proteasomes bound to MSNPN were effectively released to supernatants by excess imidazole ( Fig. 1c ), indicating that proteasome–MSNPN complex formation was mediated primarily by non-covalent His–nickel interactions, rather than non-specific adsorption or electrostatic binding. The surface zeta-potentials of nanoparticles were mildly increased from −12.60 to −6.38 mV after proteasome loading ( Supplementary Fig. 3a ), indicating reduced electrostatic repulsion among particles and stable complex formation between proteasomes and MSNPN. Moreover, nanoparticle size and hydrodynamic behaviour were comparable before and after proteasome charging ( Fig. 1d and Supplementary Fig. 3b ), suggesting that purified proteasomes were effectively loaded onto MSNPN and colloidal stability was maintained. To determine whether proteasomes bound to nanoparticles retained proteolytic activity, their ability to hydrolyse fluorogenic peptide substrate suc-LLVY-AMC was investigated. Kinetic analysis revealed comparable K M (44.4±10.7 μM proteasome–MSNPN complexes; 40.2±9.5 μM free proteasomes) and k cat (725.5±61.6 min −1 proteasome–MSNPN complexes; 427.2±51.8 min −1 free proteasomes) values (mean±s.d.) before and after complex formation ( Fig. 1e and Supplementary Fig. 4 ). These results indicated that nanoparticle-bound proteasomes remained accessible to small, peptide-based reporter substrates. We then employed a more physiologically relevant, macromolecular proteasome substrate, polyubiquitinated Sic1 PY (Ub-Sic1) [16] , to interrogate proteasome enzymatic activity. When the purified proteasomes, which retained USP14, were challenged with Ub-Sic1, Ub-Sic1 was completely degraded within 30 min ( Fig. 1f ). Proteasome–MSNPN complexes, which did not retain USP14, degraded Ub-Sic1 more rapidly than proteasomes alone, particularly at the early time points, with few Ub-chain trimming effects being observed ( Fig. 1f ). Our data may reflect the displacement of endogenous USP14 from proteasomes during the complex formation, because addition of exogenous USP14 to proteasome–MSNPN complexes delayed degradation of Ub-Sic1 ( Supplementary Fig. 5 ) [10] . However, the effect was weak, and it is likely that more than one mechanism, such as adsorption of proteasomes on MSNPN, affects catalytic activity and chain trimming effects of bound proteasomes. It will be interesting to determine whether and how USP14, endogenous or exogenous, can be utilized to regulate the functions and substrate specificity of delivered proteasomes in cells. Overall, these data indicate that it is possible to prepare non-covalent proteasome–MSNPN complexes that maintain nanoparticle colloidal stability and proteasome enzymatic activity. Proteasome–MSNPN complexes are internalized by endocytosis To determine whether MSNPN enables proteasomes to be internalized into cells, TAMRA-labeled MSNPN–proteasome complexes (compound 5 , Supplementary Fig. 6 ) were added to serum-containing culture media and incubated with HeLa cells. Cells were vigorously washed to remove free complexes and then examined by microscopy methods. Fluorescence microscopy revealed a punctate pattern for TAMRA fluorescence, consistent with localization in endocytic vesicles ( Fig. 2a ). Moreover, transmission electron micrographs (TEM) revealed the presence of nanoparticles within membrane-bounded vesicles ( Fig. 2b ). However, co-localizations between TAMRA fluorescence and lysotracker green or various endosome markers were incomplete, with both fluorescence and TEM revealing a population of nanoparticles that were free of endosomes in the cytosol ( Supplementary Fig. 7 ). At various concentrations and molar ratios, TAMRA-labelled MSNPN–proteasome complexes entered cells within 2 h after incubation and remained in the cytosol for over 96 h (data not shown). Few effects of MSNPN or proteasome–MSNPN complexes on cell viability were observed at concentrations below 300 μg ml −1 ( Supplementary Fig. 8 ) as reported in previous studies [10] , [17] , [18] . Cellular uptake of the complex appeared to be energy dependent and was processed by both caveolae- and clathrin-mediated endocytosis, as assessed by fluorescence microscopy and flow cytometry after cells were treated with proteasome–MSNPN complexes in the presence of various endocytosis inhibitors ( Fig. 2c,d and Supplementary Fig. 9 ). However, chlorpromazine (a clathrin disassembly inhibitor) more significantly delayed nanoparticle internalization than genistein (an inhibitor of caveolae-involved tyrosine kinases) or amiloride and nocodazole (inhibitors of macropinocytosis), suggesting that cholesterol-enriched lipid rafts might be utilized to engulf the relatively large-sized MSNPN [19] . 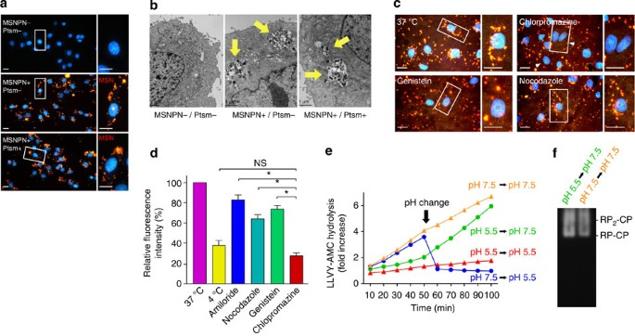Figure 2: Proteasome–MSNPN complexes are transported into cells through endocytosis. (a) Fluorescent microscope images of HeLa cells after treatment with TAMRA-labelled MSNPN alone or with proteasome–MSNPN complexes (1:50) for 24 h. Counterstained with DAPI. Bars indicate 10 μm in length. (b) As inaexcept that TEM images were taken. Arrows indicate MSNPN localized to the cytoplasm. (c) As inaexcept that proteasome–MSNPN complex uptake was blocked by various endocytosis inhibitors including genistein, chlorpromazine, and nocodazole. Bars indicate 10 μm in length. (d) Quantification of flow cytometry analysis, which measures intracellular fluorescence signals from MSNPN in the presence of endocytosis inhibitors. Bars represent the mean of percent values relative to the signal at normal conditions ±s.d. from three independent experiments. *P<0.01 (one-way analysis of variance with Bonferroni’s multiple comparison test). NS, no significance (P>0.05). SeeSupplementary Fig. 9afor the representative histogram. (e) As inFig. 1eexcept that proteasome–MSNPN complexes (1:50) under various pH conditions were used for the suc-LLVY-AMC assay. (f) The composition and activity of proteasomes before and after pH changes were determined by native polyacrylamide gel electrophoresis, followed by visualization using in-gel suc-LLVY-AMC staining. Figure 2: Proteasome–MSNPN complexes are transported into cells through endocytosis. ( a ) Fluorescent microscope images of HeLa cells after treatment with TAMRA-labelled MSNPN alone or with proteasome–MSNPN complexes (1:50) for 24 h. Counterstained with DAPI. Bars indicate 10 μm in length. ( b ) As in a except that TEM images were taken. Arrows indicate MSNPN localized to the cytoplasm. ( c ) As in a except that proteasome–MSNPN complex uptake was blocked by various endocytosis inhibitors including genistein, chlorpromazine, and nocodazole. Bars indicate 10 μm in length. ( d ) Quantification of flow cytometry analysis, which measures intracellular fluorescence signals from MSNPN in the presence of endocytosis inhibitors. Bars represent the mean of percent values relative to the signal at normal conditions ±s.d. from three independent experiments. * P <0.01 (one-way analysis of variance with Bonferroni’s multiple comparison test). NS, no significance ( P >0.05). See Supplementary Fig. 9a for the representative histogram. ( e ) As in Fig. 1e except that proteasome–MSNPN complexes (1:50) under various pH conditions were used for the suc-LLVY-AMC assay. ( f ) The composition and activity of proteasomes before and after pH changes were determined by native polyacrylamide gel electrophoresis, followed by visualization using in-gel suc-LLVY-AMC staining. Full size image The results above suggest that proteasome–MSNPN complexes are internalized through endocytic transport. To examine whether exogenous proteasomes were active and structurally intact after transport, proteasomes were incubated in an acidic pH mimicking endosomal conditions and their proteolytic activities were monitored. The proteasomal activity was substantially lower at pH 5.5 compared with at pH 7.5 ( Fig. 2e ). However, when restored to pH 7.5, proteolytic activity returned to normal levels. In contrast, lowering the pH from 7.5 to 5.5 resulted in rapid decreases in proteasome activity ( Fig. 2e ). On the basis of native gel electrophoresis and in-gel detection of suc-LLVY-AMC hydrolysis, no significant changes in proteasome composition or gating were seen after pH changes ( Fig. 2f ). Next we tested whether the MSNPN-mediated proteasome delivery could affect proteasome levels in living cells. When analysed in whole HeLa cell lysates, levels of polyubiquitins, USP14 or RP and CP subunits were little changed with proteasome–MSNPN delivery, indicating little change in overall proteasome levels or ubiquitin homeostasis ( Supplementary Fig. 10 ). However, after subcellular fractionation, significantly increased suc-LLVY-AMC hydrolysing activities were detectable in pellet fractions prepared from proteasome–MSNPN complex-treated cells relative to untreated cells ( Supplementary Fig. 11 ). These data indicate that the uptake of proteasome–MSNPN complexes into cells is accompanied by small but detectable increases in proteolytic activity. Exogenous proteasomes enhance tau protein degradation The effects of exogenous proteasome delivery on protein degradation in living cells were then investigated. Tau protein was used as substrate because it had been reported to undergo degradation via the UPS, and because this biochemical mechanism may be especially important at early stages of tauopathy and AD [8] . Cellular tau was modelled using a HEK293-derived cell line that expressed high levels of the longest central nervous system isoform of human tau (htau40) on doxycycline induction (inducible tau cell line) [20] . These cells expressed htau40 in a highly dose-dependent manner ( Supplementary Fig. 12 ), and produced slowly migrating tau species after 2 days in culture, consistent with the formation of SDS-resistant tau aggregates ( Fig. 3a ). When proteasome–MSNPN complexes were delivered to these cells, levels of overexpressed tau significantly decreased and tau protein half-life was shortened, whereas treatment with nanoparticles alone showed little effect ( Fig. 3b,c , and Supplementary Fig. 13 ). Tau mRNA levels were comparable under all treatment conditions ( Fig. 3d ), indicating that proteasome–MSNPN complexes had no effect on tau mRNA synthesis. Levels of truncated tau, which is known to be toxic and aggregative [21] , also decreased with proteasome–MSNPN treatment ( Fig. 3b ). These effects were proportional to the amount of proteasome–MSNPN complex delivered ( Fig. 3e ), but lost when free proteasomes were treated or the complexes were first inactivated by treatment with the irreversible inhibitor epoxomicin ( Supplementary Fig. 14 ). These results indicate that the enzymatic activity of delivered proteasomes is directly responsible for the degradation of overexpressed tau in these cells. 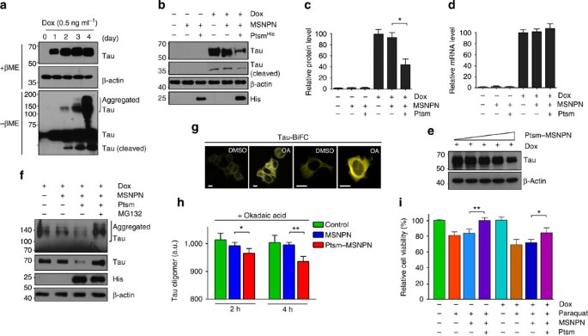Figure 3: Exogenous proteasomes enhance tau protein degradation. (a) Aggregated tau proteins and their cleaved forms were detected from the inducible tau cell line after Dox treatment (0.5 ng ml−1) for the time period indicated. Protein samples were prepared in the presence or absence of reducing reagent beta-mercaptoethanol (βME). (b) Inducible tau cell lines were treated with Dox (0.5 ng ml−1, 24 h), MSNPN (50 μg ml−1) and proteasome–MSNPN complexes (50 μg ml−1, 1:50 molar ratio, 24 h). Samples were subjected to SDS–polyacrylamide gel electrophoresis/IB. His IB is for β4 subunits of exogenous proteasomes. (c) Tau levels after treatment with Dox, MSNPN and/or human proteasomes were quantified using densitometry of film images. Bars represent the mean±s.d. from three independent experiments (n=3), *P<0.01 (analysis of variance with Bonferroni's multiple comparison test). (d) Post-translational tau regulation by exogenous proteasomes. Quantitative reverse transcription–PCR was performed using primers for tau and GAPDH (control for normalization). The values plotted are means of three independent experiments (n=3). (e) Tau degradation with graded doses of proteasome–MSNPN complexes (0, 5, 10, 25, 50 μg ml−1. 1:50 ratio). (f) As inbexcept that cells were treated with 10 μM MG132 and samples were collected under non-reducing conditions. (g) The fibrous nature and cellular localization of tau oligomers. Tau-BiFC cells were incubated with dimethyl sulphoxide (DMSO) or 30 nM of okadaic acid (OA) for 24 h. Bars indicate 10 μm in length. (h) Comparison of quantified tau oligomer levels after tau-BiFC cell lines were treated with 50 μg ml−1MSNPN and proteasome–MSNPN. Values represent the mean (±s.d.) of three independent cultures including total ~10,000 cells (SeeSupplementary Fig. 22). *P<0.05, **P<0.01. (i) Cell survival under tau induction by Dox (250 pg ml−1) and oxidative stress by paraquat, an inducer of reactive oxygen species (1 mM). Inducible tau cell lines were preincubated with Dox and paraquat for 3 h, then treated with MSNPN or proteasome–MSNPN complexes for 12 h. CCK-8 assays were performed. Values are represented as mean±s.d. (n=5). **P<0.01 (analysis of variance with Bonferroni's multiple comparison test). Figure 3: Exogenous proteasomes enhance tau protein degradation. ( a ) Aggregated tau proteins and their cleaved forms were detected from the inducible tau cell line after Dox treatment (0.5 ng ml −1 ) for the time period indicated. Protein samples were prepared in the presence or absence of reducing reagent beta-mercaptoethanol (βME). ( b ) Inducible tau cell lines were treated with Dox (0.5 ng ml −1 , 24 h), MSNPN (50 μg ml −1 ) and proteasome–MSNPN complexes (50 μg ml −1 , 1:50 molar ratio, 24 h). Samples were subjected to SDS–polyacrylamide gel electrophoresis/IB. His IB is for β4 subunits of exogenous proteasomes. ( c ) Tau levels after treatment with Dox, MSNPN and/or human proteasomes were quantified using densitometry of film images. Bars represent the mean±s.d. from three independent experiments ( n =3), * P <0.01 (analysis of variance with Bonferroni's multiple comparison test). ( d ) Post-translational tau regulation by exogenous proteasomes. Quantitative reverse transcription–PCR was performed using primers for tau and GAPDH (control for normalization). The values plotted are means of three independent experiments ( n =3). ( e ) Tau degradation with graded doses of proteasome–MSNPN complexes (0, 5, 10, 25, 50 μg ml −1 . 1:50 ratio). ( f ) As in b except that cells were treated with 10 μM MG132 and samples were collected under non-reducing conditions. ( g ) The fibrous nature and cellular localization of tau oligomers. Tau-BiFC cells were incubated with dimethyl sulphoxide (DMSO) or 30 nM of okadaic acid (OA) for 24 h. Bars indicate 10 μm in length. ( h ) Comparison of quantified tau oligomer levels after tau-BiFC cell lines were treated with 50 μg ml −1 MSNPN and proteasome–MSNPN. Values represent the mean (±s.d.) of three independent cultures including total ~10,000 cells (See Supplementary Fig. 22 ). * P <0.05, ** P <0.01. ( i ) Cell survival under tau induction by Dox (250 pg ml −1 ) and oxidative stress by paraquat, an inducer of reactive oxygen species (1 mM). Inducible tau cell lines were preincubated with Dox and paraquat for 3 h, then treated with MSNPN or proteasome–MSNPN complexes for 12 h. CCK-8 assays were performed. Values are represented as mean±s.d. ( n =5). ** P <0.01 (analysis of variance with Bonferroni's multiple comparison test). Full size image Delivered exogenous proteasomes did not affect levels of endogenous proteasome substrates Nrf2 and p53 ( Supplementary Fig. 15 ). They also did not modulate levels of tau phosphorylated at Ser 396 or Ser 199/202 ( Supplementary Fig. 16 ). These data suggest that the action of exogenous proteasomes may be limited to species that appear aberrant to the cell owing to overexpression. Consistent with this hypothesis, the low endogenous levels of tau in SH-SY5Y cells were little affected by exogenous proteasome treatment ( Supplementary Fig. 17 ). Conversely, known proteasome substrates overexpressed to high levels, such as GFPu and green fluorescent protein (GFP)-cODC, were depleted from cells by exogenous proteasome treatment, whereas GFP was not ( Supplementary Fig. 18 ). The magnitude of tau depression in inducible tau cells appeared to be partially inducer concentration dependent ( Supplementary Fig. 19 ). These results suggest that exogenous proteasomes delivered to cells may more efficiently degrade protein substrates, which impose an unusual load on the UPS, such as overexpressed tau, instead of endogenous proteasomal substrates. Future work will be required to identify distinguishing features of target proteins, such as Ub linkage specificity of tau, that underlie their differential sensitivities to proteasomal degradation. Moreover, we observed little effects of exogenous proteasomes on tau degradation when Dox concentrations were more than 3 ng ml −1 or less than 0.2 ng ml −1 . Therefore, the ‘working range’ of the delivered proteasomes is expected to be limited by the levels of overexpressed tau and its propensity to aggregate. We have no clear understanding at what magnitude pathological tau proteins accumulate in neurons as AD progresses. It will be important to determine the capacities and selectivity of exogenous proteasomes in different stages of AD and to identify the mechanistic basis of these changes. Tau aggregation is a pathological hallmark of AD. The delivery of proteasomes using MSNPN effectively delayed the formation of tau aggregates ( Fig. 3f ). This effect was independent of autophagy ( Supplementary Fig. 15 ), and was probably preceded by the accelerated proteasomal degradation of soluble tau proteins ( Fig. 3b and Supplementary Fig. 20 ). However, it was abrogated by the treatment of cells with proteasome inhibitors, which resulted in significant accumulation of both soluble tau and tau aggregates ( Fig. 3f ). In contrast, proteasome–MSNPN treatment did not alter the levels of aggregated huntingtin proteins, which are unable to be processed by proteasomes ( Supplementary Fig. 21 ) [22] . Thus, the effects of exogenous proteasomes on aggregating protein levels were restricted to UPS substrates. To visualize and quantify tau oligomerization in living cells, we utilized a tau cell line with biomolecular fluorescence complementation (BiFC) [23] . Amino-terminal and carboxyl-terminal parts of Venus proteins were independently fused to htau40, which exhibited only basal fluorescence signals under normal conditions ( Fig. 3g ). However, the fluorescence became strongly ‘turned-on’ on chemical induction of tau hyperphosphorylation, for example, by okadaic acid, consistent with consequent tau oligomerization. Similar to inducible tau cells, tau-BiFC cells treated with proteasome–MSNPN complexes showed significantly less tau aggregation compared with cells treated with MSNPN alone ( Fig. 3h and Supplementary Fig. 22 ). These results suggest that the direct delivery of exogenous proteasomes using MSNPN can delay the aggregation of tau proteins during proteotoxic conditions. Moreover, proteasome delivery significantly alleviated cytotoxicity induced by paraquat and overexpressed tau ( Fig. 3i ), showing that this method might be used to relieve proteotoxic and oxidative stress from cells. Here we report that high-molecular weight protein complexes such as human proteasomes can be directly delivered to cells using chemically modified mesoporous nanoparticles. The exogenous proteasomes retain their activity and functionality when bound to MSNPN and after they are internalized into cells through endocytosis. Increased cellular proteasome activity resulting from this treatment was tolerable to cells and did not lead to non-specific protein degradation. Importantly, cells with exogenous proteasomes showed facilitated degradation of soluble tau, delayed accumulation of tau aggregates and enhanced resistance to the proteotoxic stress mediated by tau and reactive oxygen species. Considering that silica nanoparticles are inert, nonantigenic and modifiable to be blood–brain barrier permeable [24] and that in situ regulation of proteasome biogenesis or proteasome activity is as yet to be developed, the present strategy could be an interesting alternative to regulate toxic, aggregation-prone proteins accumulated in neurons. The scope of proteasome delivery is not limited to neurodegenerative diseases, because numerous diseases are caused by toxic, misfolded, aggregation-prone proteins [25] , [26] . Thus, direct proteasome delivery may be a potentially beneficial intervention for cells under proteotoxic or oxidative stress. Materials Sources of antibodies and working dilutions are as follows: anti-tau (clone Tau-5; Invitrogen, USA, 1/10,000); anti-tau ser396 (ab109390, Abcam, USA, 1/5,000); anti-tau ser199/202 (ab4864, Abcam, 1/5,000); anti-β-actin (A1978, Sigma, 1/10,000); anti-Ub (clone P4D1, Santa Cruz, USA, 1/5,000), anti-α6 (PW8100, Enzo Life Sciences, USA, 1/3,000), anti-His (A03001, IgTherapy, Korea, 1/2,000), anti-T7 (69522, Millipore, USA, 1/5,000), anti-α3 (PW8115, Enzo Life Science, 1/5,000), anti-Rpt5 (PW8245, Enzo Life Science, 1/3,000), anti-NBR1 (sc130380, Santa Cruz, 1/2,000), anti-p62 (sc28359, Santa Cruz, 1/2,000), anti-p53 (sc1313, Santa Cruz, 1/3,000), anti-LC3 (L7543, Sigma, 1/2,000), anti-ADRM1 (PW9910, Enzo Life Science, 1/2,000), anti-USP14 (A300-920A, Bethyl Laboratories, USA, 1/2,000), and anti-GFP antibody (Enogene, USA, 1/5,000). Sources of major biochemical reagents are as follows: PS-341 (LC Laboratories, USA); epoxomicin and Ub-VS (Boston Biochem, USA); ATP (Calbiochem, USA); ubiquitin (Sigma); MG132 (Bachem); suc-LLVY-AMC (Bachem). Dulbecco’s Modified Eagle’s Medium, fetal bovine serum (FBS) and PBS (pH 7.4) were purchased from WelGENE (Korea). CCK-8 (Cell Counting Kit-8) was purchased from Dojindo Molecular Technologies (Japan) and N α ,N α -bis(carboxymethyl)- L -lysine hydrate, 3,3′-dithiodipropionic acid di( N -hydroxysuccinimide ester), chlorpromazine hydrochloride, genistein, amiloride hydrochloride hydrate, okadaic acid, doxycycline and nocodazole were purchased from Sigma. Full-size scans of original western blottings are shown in Supplementary Fig. 23 . Surface characterization of pore expanded MSN Nitrogen sorption isotherm was measured in a NOVA sorption apparatus. Surface area calculations were carried out using the Brunauer–Emmitt–Teller method, and pore size distribution was calculated according to the Barrett–Joyner–Halenda method [12] . Zeta-potential and DLS measurement Zeta-potentials and hydrodynamic sizes of MSNPN and proteasome-loaded MSNPN were measured by dynamic light scattering analysis using a Zetasizer NanoS (Malvern instruments, UK), as previously described [27] . TEM images TEM images were obtained by a LIBRA 120 EF-TEM (Carl Zeiss, Germany) at 120 kV. A drop of each MSN suspension was placed onto a Formvar-coated copper grid and stabilized with evaporated carbon film (Electron Microscopy Sciences, PA, USA). The grids were dried at room temperature for several hours before observation. To compare the TEM images of MSNPN and proteasome-loaded MSNPN, each sample was placed onto the grid and then stained with 0.5% uranyl acetate before observation. Affinity purification of the 26S human proteasome Human proteasomes were affinity purified from a stable HEK293T cell line harbouring HTBH-tagged β4 subunits. The cells were homogenized in lysis buffer (50 mM NaH 2 PO 4 (pH 7.5), 100 mM NaCl, 10% glycerol, 5 mM MgCl 2 , 0.5% NP-40) containing protease inhibitors, 5 mM ATP and 1 mM DTT, by using Dounce tissue grinders (Wheaton). Lysates were centrifuged at 10,000 g and the cleared supernatants were incubated with streptavidin agarose resin (Millipore) for 5 h at 4 °C. The beads were then incubated in TEV protease-containing elution buffer (50 mM Tris-HCl (pH 7.5), 1 mM MgCl 2 , 10% glycerol and 1 mM ATP). Endogenous Usp14 was found to be on the proteasome under these purification conditions (see Supplementary Fig. 2 ). For generating catalytically inactive proteasomes, proteasomes conjugated with MSNPN were treated with 20 μM of epoxomicin (Enzo Life science) for 2 h at room temperature. After the conjugation, epoxomicin-incubated MSNPN–proteasome (Epo–Ptsm) complexes were washed with ice-cold PBS three times. Native gel electrophoresis Native gel analysis using purified proteasomes or whole-cell lysate analysis was performed largely as previously described [10] , [28] . Samples were resolved by 3.5% nondenaturing polyacrylamide gel electrophoresis for 850 volt-hours and proteasomes were visualized using the fluorogenic substrate suc-LLVY-AMC (Bachem). After the in-gel suc-LLVY-AMC hydrolysis assay, proteins in the gel were transferred to polyvinylidene fluoride (PVDF) and subsequently immunoblotted against a CP subunit α6. Immobilizing proteasomes to MSNPN Purified proteasomes and MSNPN, using a variety of indicated molar ratios, were suspended in PBS and vigorously shaken horizontally for 2 h at room temperature. The resulting proteasome–MSNPN complexes were briefly washed three times by centrifugation at 3,000 r.p.m. The complexes were resuspended in culture media for cellular delivery. Measurement of proteasome activity on the MSNPN To see the activity of proteasomes loaded on nanoparticles, proteasome–nanoparticle complexes were prepared by incubation of 2.4 μg of proteasome with 12 μl of nanoparticle stock (10 mg ml −1 ) for 30 min at 4 °C in PBS. This was then diluted to 100 μl of final volume with assay buffer (50 mM Tris, pH 7.5, 1 mM EDTA, 1 mg ml −1 ovalbumin, 1 mM fresh ATP, 1 mM fresh DTT). Then, 10 μl of proteasome and proteasome-loaded MSNPN in assay buffer were added to a 96-well plate containing the fluorogenic substrate suc-LLVY-AMC in assay buffer. The fluorescence of AMC (ex 355/em 460) was subsequently measured. Measurement of proteasome activity from whole-cell extracts The activities of proteasomes from whole-cell extracts after the treatment of proteasome–MSNPN complexes were measured as previously described with some modifications [29] . Briefly, HeLa cells were treated for 24 h, then lysed in 50 mM NaH 2 PO 4 (pH 7.5) containing 100 mM NaCl, 5 mM MgCl 2 , 10% Glycerol, 0.2% NP-40, 1 mM ATP, 1 mM DTT and protease inhibitors. The lysates were homogenized using 26 G 3/8" syringes and centrifuged at 12,000 r.p.m. for 10 min. The resultant supernatants devoid of nanoparticles were used to measure suc-LLVY-AMC hydrolysis activity. Pellets, which include MSNPN–proteasome complexes, were resuspended in assay buffer (50 mM Tris, pH 7.5, 1 mM EDTA, 1 mg ml −1 ovalbumin, 1 mM fresh ATP, 1 mM fresh DTT) and were used to measure proteasome activities using 40 μM of suc-LLVY-AMC. The measurement was performed 37 cycles with 2 min intervals. Proteasome activity was defined as the suc-LLVY-AMC hydrolysis activity from the lysates that was inhibited by 10 μM MG132. Binding assay and imidazole elution assay The dissociation of purified proteasomes from complexes was examined by immunoblotting after brief centrifugation (1,000 g for 5 min) in the presence of imidazole (0.5 M). Unbound proteasomes in the supernatants were discarded and the pellets were either mixed with 2 × SDS sample buffer containing 2% β-mercaptoethanol or incubated with 0.5 M imidazole for 1 h. Immunoblotting was performed using anti-His antibody (IgTherapy). In vitro Ub-Sic1 degradation assay Purified human proteasomes or proteasome–MSNPN complexes (5 nM) were incubated with polyubiquitinated Sic1 PY (Ub-Sic1; 20 nM) in proteasome assay buffer (50 mM Tris-HCl (pH 7.5), 100 mM NaCl, 10% glycerol, 2 mM ATP) at room temperature for the time period indicated in the figures. Samples were mixed with 2 × SDS sample buffer, boiled for 10 min at 75 °C and subjected to immunoblotting using anti-T7 antibodies. TEM of MSNPN-treated cells Cells treated with MSNPN (80 μg ml −1 ) were fixed with 2% paraformaldehyde and 2% glutaraldehyde in 0.05 M sodium cacodylate buffer (pH 7.2) for 4 h at 4 °C. The samples were rinsed three times in 0.05 M sodium cacodylate buffer (pH 7.2) and post fixated with 1% osmium tetroxide (OsO 4 ) in 0.05 M sodium cacodylate buffer (pH 7.2) for 2 h at 4 °C. Then, they were washed with water and stained en bloc with 0.5% uranyl acetate in distilled water overnight. Samples were subsequently dehydrated in a graded ethanol series from 30 to 100%, followed by a transition to 100% propylene oxide for 15 min at room temperature twice. Infiltration was performed using a Spurr resin (mixture with ERL 4221, DER 736 epoxy resin, NSA and DMAE) series. Finally, samples were placed in fresh 100% Spurr resin in moulds and polymerized at 70 °C overnight. Ultra-thin sections were prepared with an ultramicrotome MTX (RMC, USA). Sections were loaded on a Formvar-coated copper grid, and observed by TEM (JEM 1010, Japan) at 80 kV. Kinetic analysis of proteasomes For kinetic analysis, suc-LLVY-AMC hydrolysis activity of proteasomes or proteasome–MSNPN complexes was monitored in concentration-course manners. Normalization of fluorescence intensity to AMC concentration was done using the standard curve of free AMC. The parameters K M and k cat were determined by nonlinear regression fit with a model derived from Michaelis–Menten equation using GraphPad Prism 5 (GraphPad Inc., USA). Cell culture and treatment of proteasome–MSNPN complexes Cells used in this study, including HeLa, HEK293-pre1-HTBH, HEK293-trex-htau40, tau-BiFC and HeLa-Q25/Q97-Htt-NLS were cultured in Dulbecco’s Modified Eagle’s Medium containing 4.5 g l −1 D -glucose and supplemented with 10% FBS, 100 U ml −1 penicillin and 100 g ml −1 streptomycin. Cells were maintained in a humidified incubator with 5% CO 2 at 37 °C. On the day before treatment with the proteasome–MSNPN complex, cells were seeded onto a round cover glass (φ 25Pmm, No. 1, Deckglaser, Germany). The complexes or their controls were added to adherent cells on the cover glass before the experiment, and the medium was then removed after the indicated times. Fluorescence images were obtained after cells were extensively rinsed three times with PBS to remove unbound nanoparticles. Cells expressing tau proteins were incubated with proteasome–MSNPN complexes or the same amount of MSNPN or free proteasomes. For chase analysis, HeLa cells were treated with 75 μg ml −1 cycloheximide and samples were isolated at chase times 0, 0.5, 1 and 1.5 h. For overexpression of GFPu [30] and GFP-cODC [31] , a fusion of the CL1 and ornithine decarboxylase (ODC) degrons on the carboxyl terminus of EGFP, respectively, HeLa cells were transfected with 2–4 μg of plasmid DNA in a six-well plate for 4 h using Lipofectamine 3000 (Invitrogen). Cells were lysed 36–48 h post transfection in RIPA buffer after treated with 50 μg ml −1 of MSNPN or proteasome–MSNPN complexes for 4 h. Total cell lysates were analysed by immunoblotting with anti-GFP antibody (Enogene). Cellular uptake of MSNPN with endocytosis inhibitors HeLa cells were seeded in a 12-well plate and cultured in an incubator. After 24 h, cells were treated with chlorpromazine (5 μg ml −1 ) to inhibit clathrin-dependent endocytosis, genistein (200 μM) to inhibit caveolae-dependent endocytosis or amiloride (50 μM) and nocodazole (20 μM) to inhibit macropinocytosis at 37 °C, or incubated 4 °C for 1 h in serum-free media. Cells were then incubated with 20 μg ml −1 of MSNPN for an additional 1 h under the same conditions, and washed with 2 ml of PBS three times. For quantification of nanoparticle uptake, cells were trypsinized, harvested and centrifuged at 4 °C and washed with cold PBS. Cells were resuspended in PBS containing 1% FBS and filtered. Fluorescence intensity was measured using an Aria III flow cytometer (Becton Dickinson, USA) equipped with an argon laser. Experiments were carried out in triplicate and data were shown as mean±s.d. Assessment of cell viability Cell viability was measured using the cell counting kit-8 (CCK-8) assay (Dojindo Laboratory). HeLa cells were seeded in a 96-well cell culture plate 24 h before nanoparticle treatment at a density of 1 × 10 4 cells per well. After 24 h incubation, cells were treated with varying concentrations of MSNPN, proteasome–MSNPN complexes, or small-molecule inhibitors of endocytosis. Control cells were treated with same volume of PBS. After 4 h, the media was removed, and 100 μl of serum-free media and 10 μl of CCK-8 solution were added to each well. The cells were incubated for 2 h. The optical density of formazan salt at 450 nm wavelength was measured using a microplate reader (Molecular Devices, Inc. USA), and the background absorbance of media was subtracted. The experiment was carried out in triplicate, and data were shown as mean±s.d. Quantitative RT-PCR analysis Total RNA from cultured cells was prepared using the TRIzol reagent (Invitrogen), followed by further purification through the RNeasy mini-column (Qiagen, USA) with on-column DNase I treatment. The cDNA samples were prepared by reverse transcription using Accupower RT-pre mix (Bioneer, Korea). Real-time PCR reaction was then performed using Rotor-Gene RG 3000 (Corbett Research, AU) with a diluted cDNA, SYBR qPCR master mixture (Kapa Biosystem, USA) as the reporter dye, and 10 pmol of gene-specific primers. Thermal cycling conditions were comprised of 95 °C for 3 min for enzyme activation, 40 cycles at 95 °C for 10 s, 53 °C for 15 s and 72 °C for 30 s. Each mRNA level was normalized to that of GAPDH and the values were plotted as means±s.d. of three independent experiments. Primer sequences used were as follows: for tau, forward (5′-AAGGTGACCTCCAAGTGTGG-3′) and reverse (5′-GGGACGTGGGTGATATTGTC-3′); for GAPDH, forward (5′-GAGTCAACGGATTTGGTCGT-3′) and reverse (5′-GACAAGCTTCCCGTTCTCAG-3′). Endogenous tau degradation in human neuroblastoma The SH-SY5Y human neuroblastoma cells were grown with equal amounts of minimum essential media (MEM, Welgene) and nutrient mixture Ham’s F-12 (Welgene), supplemented with 10% FBS. Proteasome–MSNPN complexes were prepared and delivered into the cells as described in ‘Immobilizing proteasomes to MSNPN’ in this method section. Cells were lysed and then subjected to immunoblotting using anti-tau antibody (Invitrogen) and anti-His antibody (IgTherapy). Tau-BiFC cell analysis A HEK293-derived stable cell line (Tau-BiFC), which constitutively expresses both the carboxyl and the amino terminus of Venus proteins independently fused with htau40, was established as recently described [23] . Tau-BiFC cells were seeded in a 96-well plate at a density of 10 5 cells per well and treated with 30 nM of okadaic acid for 24 h to accelerate tau oligomerization processes. Fluorescence images were acquired, quantified and analysed by Operetta (PerkinElmer). Statistical analysis Statistical significance of difference between various groups was determined by one-way analysis of variance followed by the Bonferroni post hoc test in most data. Differences were considered to be significant P <0.05. The Michaelis–Menten kinetic parameters were obtained by fitting the experiment data to a nonlinear regression model, using GraphPad Prism 5 (GraphPad Inc.). How to cite this article: Han, D. H. et al. Direct cellular delivery of human proteasomes to delay tau aggregation. Nat. Commun. 5:5633 doi: 10.1038/ncomms6633 (2014).